Ultraviolet and visible range plasmonics in the topological insulator Bi1.5Sb0.5Te1.8Se1.2 The development of metamaterials, data processing circuits and sensors for the visible and ultraviolet parts of the spectrum is hampered by the lack of low-loss media supporting plasmonic excitations. This has driven the intense search for plasmonic materials beyond noble metals. Here we show that the semiconductor Bi 1.5 Sb 0.5 Te 1.8 Se 1.2 , also known as a topological insulator, is also a good plasmonic material in the blue-ultraviolet range, in addition to the already-investigated terahertz frequency range. Metamaterials fabricated from Bi 1.5 Sb 0.5 Te 1.8 Se 1.2 show plasmonic resonances from 350 to 550 nm, while surface gratings exhibit cathodoluminescent peaks from 230 to 1,050 nm. The observed plasmonic response is attributed to the combination of bulk charge carriers from interband transitions and surface charge carriers of the topological insulator. The importance of our result is in the identification of new mechanisms of negative permittivity in semiconductors where visible range plasmonics can be directly integrated with electronics. Plasmons are coupled excitations of electrons in solids and electromagnetic fields, and they are responsible for the brilliant colours of some Roman vases and medieval church vitrages delivered by the colloidal suspension of gold particles in glass [1] . They are the key to nanophotonic applications and form responses of nanostructured metal surfaces and artificial metamaterial photonic structures. Plasmons can localize electromagnetic energy in the nanoscale, which is crucial for the next generation of ultra-high density optically assisted magnetic data storage technology [2] , [3] . Plasmons are exploited for enhancement of light-harvesting applications, in particular photovoltaics [4] . Plasmon resonances are used in biological sensors such as the pregnancy test [5] . Plasmon polaritons propagating on the surface are seen as a promising information carrier for ultra-compact inter-chip interconnects [6] , [7] , [8] and all-optical data processing chips [9] . However, only a narrow class of materials can support plasmons, most notably noble metals like silver and gold. In recent years, there has been a surge of research aiming to identify new plasmonic media and substantial progress has been made in the search and characterization of infrared (IR) plasmonic materials, most notably conductive oxides, nitrides and graphene [10] , [11] , [12] . The ultraviolet (UV)-visible part of the spectrum remains an extremely challenging domain for plasmonics as gold and silver have losses there, while this spectral range remains unattainable for artificially doped semiconductors and graphene [11] . The search for plasmonic metals in this spectral range is still ongoing, where aluminium surfaces as the most appealing one among them given that a controlled preparation and material analysis are accompanied to regulate the unavoidable oxidation [13] , [14] . If a low-loss plasmonic medium existed for the blue-UV part of the spectrum, this would open a plethora of important applications that could include a long-awaited metamaterial suitable for making a super-lens at optical frequency with resolution beyond the diffraction limit [15] , [16] ; a sensor sensitive to specific near-UV resonances in proteins and DNA; or an enhanced light concentrator for even further improvement of the density of optical and optically assisted data storage [17] , just to mention a few applications. In this work, using Bi 1.5 Sb 0.5 Te 1.8 Se 1.2 (BSTS) single crystals [18] , [19] , [20] , we identify a new mechanism of visible and UV plasmonic response, which is a combination of surface optical conductivity residing in a nanoscale layer of topologically protected surface states of the crystal and bulk optical conductivity related to the dispersion created by the interband transitions in the medium. In a series of optical and cathodoluminescence (CL) experiments with unstructured and nanostructured surfaces of the alloy, we show that its plasmonic properties are very well pronounced. In particular, on nanostructured metamaterial surfaces of BSTS we demonstrated plasmonic absorption peaks from 350 to 550 nm, and on grating arrays with periods from 150 to 800 nm we observed peaks of plasmonic CL in the wavelength range from 230 to 1,050 nm. Retrieved dielectric function of BSTS Plasmonics is often defined as electromagnetism at the interface between dielectrics and conductive media with negative value of the real part of dielectric permittivity ε where external field E induces displacement field D of essentially opposite direction ( D = ε E , Re{ ε }<0 and – Re{ ε }>Im{ ε }). Under such conditions, the interfaces can support highly localized oscillation and confined surface waves known as localized plasmons and surface plasmon-polariton waves [21] . Plasmons derive their name from plasma of free electrons in metals or heavily doped semiconductors [22] , [23] , [24] at interfaces of which they are often observed. Despite the huge success of modern plasmonics, the limitation of noble metals as a plasmonic material has led to the search for alternative plasmonic materials [10] , [11] . In general, there are two approaches to obtaining plasmonic behaviour at the desired frequencies. One is to heavily dope semiconductors to increase their charge carrier concentration, but this approach has been successful only up to the near-IR regime due to the difficulty in achieving the required doping level and additional losses at such a high doping level [24] , [25] , [26] , [27] , [28] , [29] . The other is to mix metals with non-metals or other metals. Titanium nitride that has been revisited recently as a promising plasmonic material for the visible and near-IR wavelengths falls into this category [10] , [30] , [31] , [32] , [33] , [34] . Apart from the bulk plasmonic materials, two-dimensional plasmonic materials such as 2D electron gas systems [35] , [36] , [37] or, recently, graphene in the mid-IR regime [38] , [39] have been attracting a huge interest due to their unusual properties such as the extreme field confinement [40] . Topological insulator is a material that behaves as an insulator in its interior but whose surface contains conducting states, meaning that electrons can only move along the surface of the material. Thus, it also falls into this category of 2D plasmonic materials [41] and the plasmons on this 2D electron gas system has been observed at terahertz frequencies recently [42] . BSTS shows a large bulk resistivity due to its ordered Te-Bi-Se-Bi-Te quintuple layers [18] , [20] in contrast to the prototypical topological insulators such as Bi 2 Se 3 and Bi 2 Te 3 . Our BSTS single crystals were synthesized by melting high-purity (99.9999%) Bi, Sb, Te and Se with molar ratio 1.5:0.5:1.8:1.2 at 950 °C in an evacuated quartz tube. The temperature was then gradually decreased to room temperature over a span of 3 weeks [19] . The BSTS single crystal was then cleaved along the (100) family of planes to a thickness of ~0.5 mm. We first investigated the optical properties of the unstructured surface by multiple-angle spectroscopic ellipsometry in the range from 200 to 1,600 nm. The measured dielectric function values before the modelling are shown in Fig. 1 as data points. The measurement results were then fitted based on the model that was successfully developed to represent low frequency conductivity of this material [19] : we assumed a material structure consisting of a bulk semiconductor with a thin metal film on top as shown in the inset of Fig. 1a . (As the BSTS crystal used in our experiments is optically thick, the bottom conducting layer can be ignored in the modelling and interpretation of our optical experiment results.) The semiconductor bulk substrate supporting the thin film was modelled using the Tauc–Lorentz [43] model that has been successfully applied to this class of materials in the past [44] , while conductivity of the topological insulator film was assumed to obey the Drude dispersion [45] . From our analysis of the spectroscopic data, we found that the best-fit parameters such as band gap of the bulk component, 0.25 eV, thickness of the topological insulator layer, d =1.5 nm and plasma and collision frequencies of Drude model, 7.5 and 0.05 eV, respectively, are close to previously reported values found for this material from the independent d.c. conductivity measurements [19] and corroborate very well with the results of ab initio calculations of dielectric functions of similar alloys [46] , [47] . 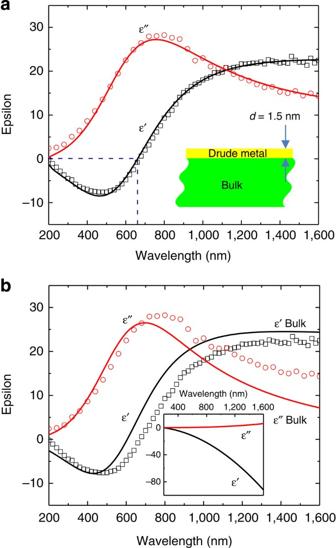Figure 1: Plasmonic properties of the BSTS topological insulator semiconductor in the visible and UV. (a) Dielectric function of the crystal retrieved from spectroscopic ellipsometry. The inset shows a sketch of the layer-on-bulk model of the crystal with a layer of topological phase of thicknessd=1.5 nm. Experimental points are presented together with the modelling data (solid lines). (b) An attempt to fit experimental data by the bulk contribution only (Tauc–Lorentz dispersion formula) show the discrepancy that is attributed to the presence of surface conductivity of topological surface state with a Drude-like dispersion (inset). We therefore conclude that the proposed layer-on-substrate material structure adequately describes optical properties of BSTS and use it for the interpretation of plasmonic response of the material (see Supplementary Table 1 and Supplementary Note 1 for details). Figure 1: Plasmonic properties of the BSTS topological insulator semiconductor in the visible and UV. ( a ) Dielectric function of the crystal retrieved from spectroscopic ellipsometry. The inset shows a sketch of the layer-on-bulk model of the crystal with a layer of topological phase of thickness d= 1.5 nm. Experimental points are presented together with the modelling data (solid lines). ( b ) An attempt to fit experimental data by the bulk contribution only (Tauc–Lorentz dispersion formula) show the discrepancy that is attributed to the presence of surface conductivity of topological surface state with a Drude-like dispersion (inset). Full size image Negative permittivity of BSTS is clearly seen between the wavelengths, 200 and 670 nm ( Fig. 1a ). It is instructive to observe that the negative epsilon regimes in this spectral range are characteristic to both components of the structure, the Drude layer and underlying bulk semiconductor, as shown in Fig. 1b . However, the bulk contribution alone is not sufficient to explain dielectric properties of the material especially in the long wavelength regime as illustrated in Fig. 1b . The topologically protected surface charge carriers are forming the response of the top metallic layer: if such conductivity would exist in the bulk medium, plasmonic properties of such hypothetical material would be better than that of any known plasmonic material in this spectral range (see Supplementary Figs 1 and 2 and Supplementary Note 2 ). Here we see that even a thin layer of the topological phase has a profound impact on plasmonic response of the structure even when placed on a lossy substrate. Our analysis of the ellipsometry data shows that it adds up to 8% to the reflectivity of the nanostructured surface (see Supplementary Fig. 3 and Supplementary Note 3 ). The bulk plasmonic response here largely originates from the interband absorption dispersion in this material, not from the bulk free carriers. Its origin is similar to that of the negative dielectric permittivity area at the higher frequency wing of the isolated absorption peak that corresponds to the peak in joint density of states in case of semiconductor. It can be understood as an inevitable consequence of the Kramers–Kronig relations that link the real and imaginary parts of permittivity near a strong absorption peak, as has been observed near IR phonon lines [48] , [49] . Negative permittivity due to interband transitions has been theoretically predicted for a similar material of Bi 2 Se 3 in electronic structure calculations within the density function theory based on full potential linearized augmented plane wave and local orbitals [46] , [47] . However, to our knowledge, BSTS represents the first example of material where negative permittivity due to interband electronic absorption is seen at the optical frequencies experimentally. We argue that negative permittivity due to the strong interband absorption can only be seen in semiconductors where background or zero-frequency permittivity is small enough to be overcome by negative resonant contribution and BSTS is the first known example. Polarization-dependent absorption of nanostructures on BSTS To verify the plasmonic behaviour of BSTS in nanostructures, we manufactured a series of metamaterials, nano-slit antenna arrays with linear grooves cut into the surface of the crystal, and gratings on the crystal surface using focused ion-beam milling ( Fig. 2 ). In the nano-slit antenna array, the slit length D was varied from 100 to 400 nm and the period of the slit arrays (unit cell size, UC) was kept at 300 nm for D =100–225 nm and UC =1.5 D for D =250–400 nm. The fabricated nano-slits’ profile is close to V-shape, as shown in Fig. 2b . 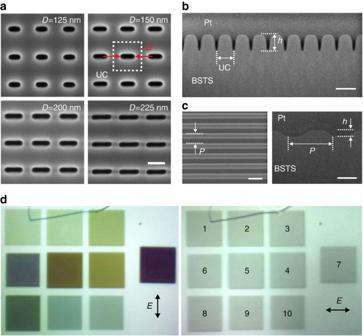Figure 2: Nanostructured topological insulator: metamaterial and grating. (a) Scanning electron microscopic (SEM) images of the nano-slit array metamaterials with nominal lengths of the slits ofD=125, 150, 200 and 225 nm. The unit cell (UC) size is 300 × 300 nm. Scale bar, 200 nm. (b) Cross-section of the array perpendicular to the nano-slit shows the slit profile with depth ofh=300 nm. Platinum layer was deposited for protection during sectioning. Scale bar, 400 nm. (c) SEM image top view (left) and cross-section view (right) of a grating with periodP=500 nm and depthh=70 nm. Scale bars, 500 nm (left), 200 nm (right). (d) Plasmonic colours can be seen in optical images of nano-slit array with polarized light illumination perpendicular to the slits (left) and are not seen for parallel polarization (right). Light polarization is indicated by the arrow. Individual sample have sizes of 40 × 40 μm. The number 1 to 10 on right figure annotate lengths of the nano-slits in the arrays: 1↔100 nm, 2↔125 nm, 3↔150 nm, 4↔175 nm, 5↔200 nm, 6↔225 nm, 7↔250 nm, 8↔300 nm, 9↔350 nm and 10↔400 nm, respectively. Figure 2: Nanostructured topological insulator: metamaterial and grating. ( a ) Scanning electron microscopic (SEM) images of the nano-slit array metamaterials with nominal lengths of the slits of D =125, 150, 200 and 225 nm. The unit cell (UC) size is 300 × 300 nm. Scale bar, 200 nm. ( b ) Cross-section of the array perpendicular to the nano-slit shows the slit profile with depth of h= 300 nm. Platinum layer was deposited for protection during sectioning. Scale bar, 400 nm. ( c ) SEM image top view (left) and cross-section view (right) of a grating with period P =500 nm and depth h =70 nm. Scale bars, 500 nm (left), 200 nm (right). ( d ) Plasmonic colours can be seen in optical images of nano-slit array with polarized light illumination perpendicular to the slits (left) and are not seen for parallel polarization (right). Light polarization is indicated by the arrow. Individual sample have sizes of 40 × 40 μm. The number 1 to 10 on right figure annotate lengths of the nano-slits in the arrays: 1↔100 nm, 2↔125 nm, 3↔150 nm, 4↔175 nm, 5↔200 nm, 6↔225 nm, 7↔250 nm, 8↔300 nm, 9↔350 nm and 10↔400 nm, respectively. Full size image The plasmonic response of the fabricated nano-slit metamaterials and gratings were studied by measuring their reflection spectra R ( λ ) and their corresponding absorption spectra A ( λ )=1– R ( λ ) for two incident polarizations perpendicular and parallel to the nano-slits ( Fig. 3a,b ). The nano-slit arrays clearly exhibited plasmonic colours for light polarized perpendicularly to the slits, as can be seen in the optical microscope images (see Fig. 2d ). A profound resonance in plasmonic absorption can be seen for this polarization ( Fig. 3a ). Indeed, if a wire dipole is resonant for light polarized along the dipole, according to the Babinet principle, slits in the conductive surface, the ‘anti-dipole’, will be resonant for perpendicular polarization. Here, the resonant wavelength increases monotonously with the length of the slit as can be seen in Fig. 3c . As expected, no plasmonic resonance can be found in the polarization along the slits (see Fig. 3b ). On all graphs presented in Fig. 3b , an absorption peak near 400 nm is seen. It is due to a feature in the bulk interband absorption and is also observed from unstructured surfaces. For short slits, the plasmonic peaks overlap with the interband absorption feature and became distinct for D >175 nm. Full three-dimensional Maxwell calculations of the reflectivity spectra obtained on the basis of ellipsometry data strongly corroborate with experimental results (see Supplementary Note 3 ). In the numerical calculations, slits were modelled as in Fig. 3d and their shape is much more difficult to reproduce for shorter slits, than for longer slits. The fabrication process finesse is limited by the spot size of the focused ion beam (~16 nm) and this explains some mismatch between the simulation and experiment seen for shorter slits in Fig. 3c . 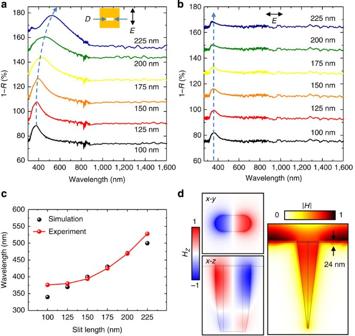Figure 3: Plasmonic properties of nano-slit array metamaterials fabricated on topological insulator semiconductor. (a) Absorption spectra, 1−R, of various nano-slit arrays with lengthsDfrom 100 to 225 nm for light polarized perpendicular to the slits nano-slits and (b) parallel to nano-slits. Spectra are offset for clarity. (c) Peak wavelength of the absorption resonance for various slit lengths increases with the slit lengthD.(d) Maxwell modelling of theHz- and |H|- field distribution in the slit length of 175 nm at the resonance wavelength of 430 nm indicates that light is localized in the surface layer of thicknessx~24 nm (incident light polarization is perpendicular to the nano-slit). Different cross-sections of the slit are shown. Figure 3: Plasmonic properties of nano-slit array metamaterials fabricated on topological insulator semiconductor. ( a ) Absorption spectra, 1− R , of various nano-slit arrays with lengths D from 100 to 225 nm for light polarized perpendicular to the slits nano-slits and ( b ) parallel to nano-slits. Spectra are offset for clarity. ( c ) Peak wavelength of the absorption resonance for various slit lengths increases with the slit length D. ( d ) Maxwell modelling of the H z - and | H |- field distribution in the slit length of 175 nm at the resonance wavelength of 430 nm indicates that light is localized in the surface layer of thickness x ~24 nm (incident light polarization is perpendicular to the nano-slit). Different cross-sections of the slit are shown. Full size image In another series of experiments, we investigated the optical response and CL spectra of gratings fabricated on the surface of topological insulator. The periods P of gratings were chosen for their diffraction peaks to be located at different wavelengths from the UV to visible parts of the spectrum. The width of the grating ridge was maintained to be the half the grating period P . Deep gratings (70 nm) with the periods, P from 200 to 1,500 nm, were fabricated on the surface of a bulk BSTS crystal as shown in Fig. 2c . The plasmonic response was found in the gratings when they were illuminated with the polarization perpendicular to the grating rulings as shown in Fig. 4a . In contrast to the featureless absorption spectra for the parallel polarization, the formation and evolution of 1st and 2nd-order peaks were clearly seen for the perpendicular polarization in the wavelengths range between 350 and 670 nm. Moreover, peaks were also visible for wavelengths longer than 670 nm. 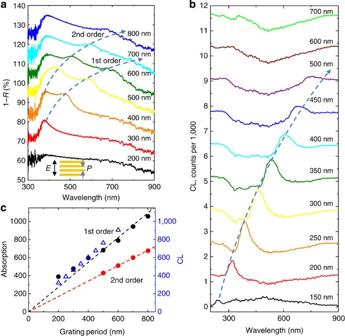Figure 4: Plasmonic properties of gratings fabricated on topological insulator semiconductor. (a) Absorption spectra of one-dimensional gratings with pitchPfrom 200 to 800 nm, in 100-nm steps for the incident polarizations perpendicular to the grating. (b) CL spectra of the gratings with period from 150 to 700 nm. (c) Peak wavelength of the absorption and CL resonances for various periods of the grating (triangles-CL data; circles-absorption data). Linear fits to the absorption data points of the formAxare shown (dashed lines), whereA=1.37 and 0.85 for 1st- and 2nd-order peaks, respectively. Figure 4: Plasmonic properties of gratings fabricated on topological insulator semiconductor. ( a ) Absorption spectra of one-dimensional gratings with pitch P from 200 to 800 nm, in 100-nm steps for the incident polarizations perpendicular to the grating. ( b ) CL spectra of the gratings with period from 150 to 700 nm. ( c ) Peak wavelength of the absorption and CL resonances for various periods of the grating (triangles-CL data; circles-absorption data). Linear fits to the absorption data points of the form Ax are shown (dashed lines), where A =1.37 and 0.85 for 1st- and 2nd-order peaks, respectively. Full size image CL spectroscopy of nanogratings These results should be compared with our CL data that have also been successfully used in the past to identify plasmonic response [50] . The gratings were excited with electron beam (waist diameter ~50 nm; electron energy 40 keV; beam current ~10 nA) of a scanning electron microscope. The electron beam was raster scanned on an area of about 10 × 10 μm of each grating. Figure 4b shows the normalized CL spectra from each grating where the CL from the unstructured crystal surface was subtracted. Peaks in the range from 230 to 1,050 nm can be observed. The emission peaks and their red-shift with increase of the grating period are clearly observed. Importantly, CL peaks’ positions accurately match that of the absorption peaks emphasizing their common plasmonic nature of the responses ( Fig. 4c ). Here, we argue that the observation of the CL peaks for wavelengths beyond 670 nm, that is, beyond the range of wavelengths where dielectric permittivity of the bulk is negative, is a clear evidence of plasmonic contribution of the topological surface conducting state. To further illustrate the contribution from the surface conducting state, the same CL experiment was conducted on another set of gratings with constant period P but variable width of the grating ridge, w . Since the plasmon wavelengths of the topological surface conducting layer and bulk layer are drastically different (wavelength of the surface plasmon polariton on the topological surface conducting layer is about hundred times shorter than that on the surface of the semiconductor), we shall expect that optical response of the gratings with ridge that is much narrower than the plasmon wavelength should be dominated by the plasmonic response of the topological surface conducting layer, in particular outside of the bulk negative permittivity regime. This is exactly what we saw in our additional experiments (see Fig. 5 ). 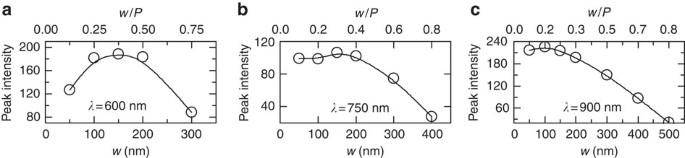Figure 5: Field enhancement observed in CL peaks outside negative epsilon regime. Peak intensities of CL as a function of the filling factor of the grating,w/P, for grating periods, (a) 400, (b) 500 and (c) 600 nm. The ridge width was varied from 50 to 500 nm. Figure 5: Field enhancement observed in CL peaks outside negative epsilon regime. Peak intensities of CL as a function of the filling factor of the grating, w/P , for grating periods, ( a ) 400, ( b ) 500 and ( c ) 600 nm. The ridge width was varied from 50 to 500 nm. Full size image The peak intensity of CL peaks was monitored as the filling factor of grating, w/P , was varied between 0 to 1 for fixed grating periods of 400, 500 and 600 nm. Peak CL wavelengths of those gratings were at 600, 750 and 900 nm, respectively. For 400 nm period gratings, peak is located at 600 nm within the epsilon-negative regime, but, for gratings with period of 500 ( Fig. 5b ) and 600 nm ( Fig. 5c ), peaks are located at 750 and 900 nm outside of the bulk epsilon-negative regime. Without a geometry-dependent plasmonic field enhancement mechanism, the peak CL intensity would simply depend on the diffraction efficiency of the grating, which has its optimum at w/P ~0.5 and falls down as this filling factor becomes closer to 0 or 1. For the 400 nm period gratings with peak at 600 nm, the CL peak intensity clearly follows the diffraction efficiency curve as the filling factor is varied ( Fig. 5a ), indicating that bulk plasmonic effects dominate in the response. However, for gratings with period of 500 ( Fig. 5b ) and 600 nm ( Fig. 5c ) whose peaks are located at 750 and 900 nm outside of the bulk epsilon-negative regime, the decrease of the grating ridge width, w , does not lead to a fall in the diffraction intensity: even gratings with very narrow ridges, down to 50 nm show profound diffraction. This remarkable robustness of diffraction can only be explained by a prominent presence of plasmonic enhancement mechanism in narrow ridges. It can only be provided by a plasmonic medium with the wavelength of the surface plasmon that is much shorter than that of free-space wavelength at 750 nm and 900 nm. (For example, plasmon wavelengths of topologically protected surface carriers [51] and bulk carriers are 0.83 and 597 nm at free-space wavelength of 600 nm, see Supplementary Note 4. ) In the material sample under study, this can only be explained by the plasmonic response of the topological surface conducting layer with the plasmon wavelength that is short enough to form localized plasmonic resonances in narrow, deeply subwavelngth ridges. We argue that this CL data unambiguously corroborate with our ellipsometry data regarding the presence and substantial role of the topologically protected surface layer in the optical response of the material. In summary, we have demonstrated the plasmonic behaviour of a topological insulator semiconductor, BSTS, at optical frequencies. It resulted from a combination of contributions from the topologically protected surface conducting state and a strong dispersion due to the interband transition. In contrast to the prejudice that plasmonic behaviour is not attainable around the interband transition both in semiconductors and metals, the optical and electron beam excitation of the material demonstrated the existence of the plasmonic response in such a case. Such bulk plasmonic properties could also be found in more simple semiconductors. Further band engineering might be able to tune the negative epsilon regime with moderate loss to the longer wavelengths than that of BSTS reported in this manuscript. However, the big advantage of topological insulators is that they provide additional, robust way of achieving optical Dirac plasmons compared with those in graphene or other 2D materials. We believe that the importance of our results is in the identification of new class of materials with high-frequency plasmonic response where plasmonic functionality can be directly integrated with electronics thanks to the semiconductor nature of the material. Sample fabrication Arrays of nano-slit antennas and gratings were patterned on the top surface of a 0.5 mm thick BSTS crystal with a focused ion-beam system (FEI Helios 600 NanoLab). The lateral dimension of each fabricated sample was 40 × 40 μm. Optical measurements The reflection spectra of the nano-slit antenna arrays and gratings were recorded using a microspectrophotometer (CRAIC QDI2010). The optical microscope image of Fig. 2d was taken via the microspectrophotometer. The dielectric function of the bulk BSTS crystal was obtained with a spectroscopic ellipsometer (Horiba UViSEL2, spot size ~1 × 1.2 mm). CL measurements The CL spectra of nanostructures were acquired in a scanning electron microscope (Camscan) equipped with a UV–visible spectrometer and a liquid nitrogen cooled charge-coupled device detector. The electron beam excitation (spot diameter ~50 nm; electron energy 40 keV; beam current ~10 nA) was carried out by raster scanning on the area of 10 × 10 μm. How to cite this article: Ou, J.-Y. et al. Ultraviolet and visible range plasmonics in the topological insulator Bi 1.5 Sb 0.5 Te 1.8 Se 1.2 . Nat. Commun. 5:5139 doi: 10.1038/ncomms6139 (2014).